Cultivation-based multiplex phenotyping of human gut microbiota allows targeted recovery of previously uncultured bacteria The human gut microbiota is linked to a variety of human health issues and implicated in antibiotic resistance gene dissemination. Most of these associations rely on culture-independent methods, since it is commonly believed that gut microbiota cannot be easily or sufficiently cultured. Here, we show that carefully designed conditions enable cultivation of a representative proportion of human gut bacteria, enabling rapid multiplex phenotypic profiling. We use this approach to determine the phylogenetic distribution of antibiotic tolerance phenotypes for 16 antibiotics in the human gut microbiota. Based on the phenotypic mapping, we tailor antibiotic combinations to specifically select for previously uncultivated bacteria. Utilizing this method we cultivate and sequence the genomes of four isolates, one of which apparently belongs to the genus Oscillibacter ; uncultivated Oscillibacter strains have been previously found to be anti-correlated with Crohn’s disease. The human gut microbiota is a diverse microbial environment consisting of mostly anaerobic bacteria containing up to 10 12 cells per gram of faecal matter [1] . The links with human disease [2] , [3] , [4] and other health concerns such as obesity [5] , [6] have made it an important area for research. Increasing concerns about antibiotic resistance have also led to further study in the human gut as it is an ideal environment for acquisition and transfer of resistance genes to occur [7] , [8] , [9] , [10] . New advances in culture-independent methodologies to study microbial communities have revolutionized how we study the human microbiome [1] , [11] , but in the process use of culture-based approaches has declined. While culture-independent methods can address a range of complex questions [12] , [13] , these approaches cannot make the definitive links to bacterial physiology that culturing does. Consequently, there is an increasing interest in improving culturing techniques for studying the gut microbiota. Advances in culturing techniques include encapsulation of bacteria into microdroplets [14] , [15] , diffusion chambers simulating the natural environment of the samples [16] , [17] , microfabricated cultivation chips [18] and design of more effective culture media [19] , [20] , [21] with high-throughput identification of the cultured bacteria [22] . Furthermore, there have been several studies looking at the effect of using alternative solidifying agents to agar [20] , [21] . The use of combinations of media has also allowed sampling of a more diverse collection of bacteria. Indeed, a recent study utilizing 212 different culturing conditions retrieved 340 bacterial species from three human stool samples [23] . In spite of recent advances, it remains widely believed that our ability to culture the human gut microbiota is far from comprehensive and relies on complicated techniques that cannot be readily implemented in most laboratories. Consequently, there remains a need for relatively simple procedures to cultivate and characterize the human gut bacterial community. Here, we combine novel cultivation conditions with high-throughput sequencing to identify conditions that allow representative cultivation and multiplex phenotypic profiling of the gut microbiota, allowing cultivation of important previously uncultivated species. Anaerobic culturing recovers substantial part of live cells To identify optimal anaerobic cultivation conditions for cultivating the human gut microbiota, we tested the growth of bacteria from faecal samples on 10 different solid media. These media were chosen to represent a range of nutrient concentrations and several had previously been shown to have good potential for recovery of gut bacteria [22] , [24] , [25] . The goal was to try to more closely represent the conditions in the gut; hence, a careful consideration of media components was undertaken ( Supplementary Discussion ). The growth was monitored over 7 days and it was observed that the colony count levelled out by day 3 for the majority of media ( Supplementary Fig. 1 ). One of the lower nutrient media had pronounced growth between days 5–7, suggesting continued growth with increased incubation times. The lower nutrient media (GM1 and GM2 (M9 agar and gellan)), GM3 (GMM agar) and GM4 (GMM gellan) media (see Supplementary Methods for complete media descriptions) also tended to have overall lower plate counts. About half of the tested media had roughly the same (10 10 ) final colony counts, although the growth patterns varied by medium. The GM7 (modified GAM agar) medium had the highest overall plate counts. Notably, a difference in solidifying agent (agar versus gellan) affected the growth on all media ( Supplementary Fig. 1 ). It is commonly believed that only a minor part of the gut microbiota can be cultivated using any specific cultivation condition [26] , [27] . To assess the extent to which the colony counts correlated with the number of live cells present in our samples, we determined the fraction of live cells by microscopy (Methods) in parallel to cultivation using three independent samplings of two unrelated human adult volunteers. By determining the viable cells counts over time we hoped to establish that similar counts could be repeated in the same individual and determine if there was a large variability between individuals. Notably, the percentage of culturable cells (plate counts/viable cell counts) had a modest variability over time and varied between 30 and 40% for the two volunteers ( Fig. 1a ). This demonstrates that a substantial fraction of the viable bacteria in the gut microbiota can form colonies under these conditions. In contrast, the viable cells and culturable cells only represented 44% and up to 17% of the total cells, indicating the presence of dead or non-viable cells in the sample. 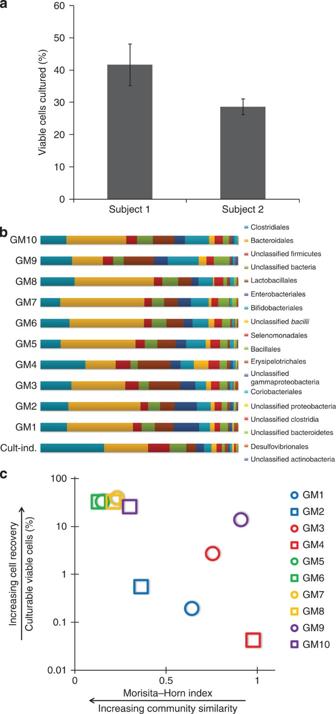Figure 1: Effectiveness of culturing conditions for recovery of human gut bacterial community. (a) The percentage of viable cells that we were able to culture. It was determined by dividing the GM7 plate counts by the trypan blue viable cell counts. The viable cells cultured were calculated for faecal samples obtained from two human subjects over three time points to show reproducibility across time and subjects. (b) An order-level taxonomic comparison of all tested media and the culture-independent (Cult-Ind.) sample based on tag abundance (Sample D1-T1). The order of the taxa is by abundance of the culture-independent sample. Bacterial taxa represented by less than five sequences for all samples are not displayed. (c) An assessment of each culture media’s effectiveness for the recovery of the human gut bacterial community. The smaller the Morisita–Horn dissimilarity index (range from 0 to 1) and larger the percentage of recovered viable cells, the better the culture media represented the culture-independent community. Thexaxis represents the Morisita–Horn index and theyaxis indicates the percentage of viable cells cultured on each media (Sample D1-T1). Figure 1: Effectiveness of culturing conditions for recovery of human gut bacterial community. ( a ) The percentage of viable cells that we were able to culture. It was determined by dividing the GM7 plate counts by the trypan blue viable cell counts. The viable cells cultured were calculated for faecal samples obtained from two human subjects over three time points to show reproducibility across time and subjects. ( b ) An order-level taxonomic comparison of all tested media and the culture-independent (Cult-Ind.) sample based on tag abundance (Sample D1-T1). The order of the taxa is by abundance of the culture-independent sample. Bacterial taxa represented by less than five sequences for all samples are not displayed. ( c ) An assessment of each culture media’s effectiveness for the recovery of the human gut bacterial community. The smaller the Morisita–Horn dissimilarity index (range from 0 to 1) and larger the percentage of recovered viable cells, the better the culture media represented the culture-independent community. The x axis represents the Morisita–Horn index and the y axis indicates the percentage of viable cells cultured on each media (Sample D1-T1). Full size image Cultivation allows representative sampling of gut microbiota To assess the diversity of microorganisms capable of growing under our different cultivation conditions relative to those identified using culture-independent methods, we determined the phylogenetic diversity of bacteria grown on each of our different cultivation media. We first combined multiple dilutions from each media in equal proportions to better sample the microbes capable of growing on each media (Methods). Our goal was to identify bacteria that were culturable at some point during the 7-day growth period. We are confident that most colonies did not grow as co-cultures, as visual observation showed most colonies did not appear to touch (Methods), so we do not anticipate that they represented a substantial proportion of the population. Colonies were resuspended from solid media and DNA was extracted. Previous work from Goodman et al. [22] indicated that inoculum from non-viable or non-growing cells does not represent more than 2% of sequences recovered from scraping plates (sample diluted 10,000-fold). Most cells we recovered were from samples diluted 100,000 to 1,000,000-fold, further decreasing the likelihood of DNA persisting through the incubation period from non-growing cells. The V6 region of the 16S rRNA was amplified and sequenced to yield phylogenetic profiles for each of the growth conditions. To remove the noise from errors in sequencing, we applied a filtering step during the initial sequence processing as previously suggested for Illumina data [28] (Methods). After filtering, each unique sequence (100% similarity) was considered a phylogenetic tag and subsequent analyses are based on these tags. A graph of the taxonomic classifications (order level) and tag counts of each of the media and culture-independent sample highlights the differences in taxonomic representation between the samples. It was observed that 66–81% of order-level and 50–71% of family-level taxonomic groups from the total faecal sample were recovered on the tested media ( Fig. 1b ). If all media were combined, a total of 95% of order-level and 88% of family-level taxonomic groups were recovered. It was also observed that changing a solidifying agent increased selection (relative sequence abundance) for certain taxa ( Supplementary Fig. 2a ). Lactobacillaceae increased in GM4 (gellan) compared with GM3 (agar; Supplementary Fig. 2b ) as opposed to an increase of Enterococcaceae in GM3 (agar) compared with GM4 (gellan; Supplementary Fig. 2c ). In other cases, the nutritional components (media composition) caused a selection as observed for Actinobacteria and Enterococcaceae , which are enriched in the GM9 (diluted modified GAM agar) and GM10 (diluted modified GAM gellan) as compared with most other media ( Supplementary Fig. 2d ). Ninety-three of the tags (54.4% of unique tags) from the culture-independent sample were not represented in any culture media ( Supplementary Data 1 ). However, these tags made up only a minority of the total sequences (15.8%) indicating many were of low abundance. None of these low-abundance tags represented more than 2% of the uncultivated community. As total bacterial cells in the gut are known to reach 10 12 Colony-forming units (CFU) g −1 , dead cells that would be unable to be cultured likely represent some of the discrepancy between the methods. However, since distinct bacterial populations are unlikely to be composed of a single cell, we would expect that most bacteria have viable representatives within the sample. While the observance of tags unable to be recovered by culturing was anticipated, we were able to recover tags that represented 84% of sequences ( Supplementary Data 2 ) in the gut microbiota (recovered in uncultivated sample). Notably, these tags represented the majority of sequences in the uncultivated sample. Recovery from individual media ranged from 68 to 78% (sequences). We also observed the recovery of 113 tags in culture that were not found in the culture-independent sample ( Supplementary Data 3 ). The identity of these tags varied between media and originated from a variety of taxonomic groups. Many of these tags were selected for by multiple media and could be found in varying abundances. Not all of them appeared to be of very low abundance. Indeed, a number of Clostridia / Clostridium tags were among the culture-only isolates. Clostridia are well-known endospore formers that can be difficult to lyse in spore form [29] . These endospores may form during passage from the body, but sporulate into vegetative cells due to more favourable culture conditions making their recovery more likely. Other taxa poorly recovered in the total faecal sample include Staphylococcaceae and Enterococcaceae , whose thick gram-positive cell walls can also present a barrier to extraction [30] , [31] . We cannot rule out the possibility that some variation arose due to variation in technical replicates and because slightly different extraction methods were used for the faecal samples versus the cultured samples. The results highlight that while both culture-dependent and independent methods can broadly capture the same bacterial constituents, they also select for distinct subsets of the gut microbiota. We then quantified the similarity between the tags obtained from different cultivation media to the community as determined using a culture-independent approach using the Morisita–Horn index, which measures the dissimilarity in community structure. We chose this comparative index because we are not only interested in maximizing the recovery of tags shared with the uncultivated sample, but also in preserving overall community structure. A similar community structure could indicate that growth conditions more closely represent what is found in the gut, better representing the microbiota’s natural environment. We found that media GM5 (GAM agar), GM6 (GAM gellan), GM7 (modified GAM agar) and GM8 (modified GAM gellan) had average Morisita–Horn indices of 0.18 (Morisita–Horn index can range from 0 to 1), which demonstrates that the overall community architecture is well represented in these media. This is supported by biological replicates of the culture-independent sample showing Morisita–Horn indices of 0.12, while technical replicates had Morisita–Horn indices of less than 0.04 indicating homology in PCR replicates. An optimal media would have a low Morisita–Horn index relative to the cultivation-independent community and a high percentage recovery of live cells. Notably, media GM5, GM6, GM7, GM8 and GM10 closely clustered to show good recovery, while the remaining media were scattered along the graph highlighting the factors causing their divergence from the culture-independent sample ( Fig. 1c , Supplementary Fig. 3 ). The GM4 media was clearly the worst media, while several nutritionally similar media (GM5, GM6, GM7 and GM8) were the best. The GM7 had a slightly higher recovery of viable cells compared with the other similarly composed media (GM5, GM6 and GM8) while maintaining a high community structure similarity to the culture-independent sample. Further discussion on the cultivation and media is available in Supplementary Discussion . Since human gut microbiomes across individuals and geography are highly variable [32] , the same effectiveness of these media may not be reflected across all samples tested. We suggest an application of this methodology to determine media appropriate to specific studies. To show that similar recovery could be repeated across several samples, we applied our GM7 media to compare culture-dependent and independent samples ( Supplementary Fig. 4 ). Our results demonstrate that the recovery of taxonomic groups was repeatable both over time in the same subject and between multiple subjects. Cultivation-based multiplex antibiotic tolerance phenotyping Using high-throughput sequencing of the cultured community, we were able to demonstrate that a good representation of the human gut microbiota can be cultivated on several of our media. The use of cultivation to survey a bacterial community provides us with the advantage of being able to link phenotypic characteristics to a particular taxa, which cannot be as definitively characterized by culture-independent methods. This method of phenotyping via culturing can be easily multiplexed to simultaneously look at specific phenotypic characteristics within a range of taxa within a given microbial community, which we term cultivation-based multiplex phenotyping. To demonstrate this, we mapped the antibiotic tolerance phenotypes of the human gut microbiota, which demonstrates functionality (phenotypic tolerance) rather than only observed genotypes [33] . A faecal sample from a healthy volunteer that had been antibiotic free for the preceding year was tested against 16 different antibiotics ( Supplementary Table 1 ). The antibiotic concentrations targeted 2 × the minimum inhibitory concentrations (MICs; average) of commensal gut bacteria (mostly Bacteroidetes, Enterococcaceae, Enterobacteriaceae and Lactobacillus ) based on Eucast data ( http://mic.eucast.org/Eucast2/ ). These antibiotic concentrations are not necessarily clinically relevant, but demonstrate how multiplex culture-based phenotyping can be applied to study microbial phenotypes. Without antibiotic selection we recovered 1.7 × 10 10 CFU g −1 , while the presence of antibiotics reduced the recovery to 5.1 × 10 7 –1.5 × 10 10 CFU g −1 , except for the chloramphenicol plates, which did not support growth ( Supplementary Fig. 5 ). The antibiotics clindamycin and metronidazole had the lowest prevalence of tolerance phenotypes in the sampled gut microbiota varying between 0.3% and 1.1%. This is consistent with their common use to target anaerobic bacterial infections [34] . In contrast, gentamycin had the highest prevalence of tolerance phenotypes (91.4%), which is consistent with previous reports highlighting its reduced capability to inhibit growth of anaerobic and facultative anaerobic bacteria under anaerobic conditions [35] , [36] . In general, tolerance phenotypes towards beta-lactams (ampicillin, cefepime, cefotaxime, cephalexin, cefuroxime, dicloxacillin and piperacillin) were high; on average, 33% of the recovered taxa (tags) were able to grow in the presence of various beta-lactam antibiotics (calculated by determining (average counts on beta-lactam plates)/(control plate counts)). To assess which tags were retrieved under different antibiotic selective pressures, the two dilutions above the countable plate (two replicates per dilution) were collected and sequenced after 5 days of incubation at 37 °C (see Methods). The tags were taxonomically classified ( Supplementary Data 4 ) and a heat map was created in R to visualize the data ( Fig. 2a ). These mapped tags represent those that were also recovered on control plates (bacteria making up the majority of the gut community). This data provides a representative view of how antibiotic tolerance phenotypes are distributed across taxonomic groups in the microbiota ( Fig. 2b–e ). A mapping of all tags recovered as adjusted by plate count recovery ( Supplementary Fig. 6 ) allows a more accurately proportional representation of the tags recovered on each antibiotic. 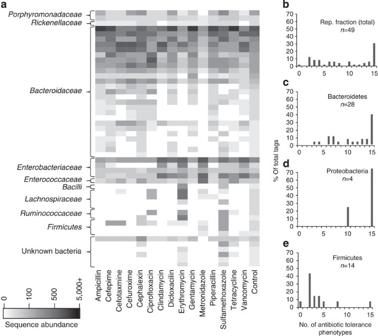Figure 2: Antibiotic tolerance distributions in majority gut bacterial populations. (a) The taxonomic classifications and proportions of tags representing the majority of cells within the gut community and their associated antibiotic tolerance phenotypes. The representative majority consists of the tags that were also recovered on the control plates. The tags are sorted by taxonomy and the highest level of classification was reported. (b) The number antibiotic tolerance phenotypes associated with each tag found in the representative majority of gut bacterial communities. (c–e) The number of tolerance phenotypes found per tag split into the (c)Bacteroidetes, (d)Proteobacteriaand (e)Firmicutesphylums. The number of tags associated with each phylum is also reported (n)=x. Figure 2: Antibiotic tolerance distributions in majority gut bacterial populations. ( a ) The taxonomic classifications and proportions of tags representing the majority of cells within the gut community and their associated antibiotic tolerance phenotypes. The representative majority consists of the tags that were also recovered on the control plates. The tags are sorted by taxonomy and the highest level of classification was reported. ( b ) The number antibiotic tolerance phenotypes associated with each tag found in the representative majority of gut bacterial communities. ( c – e ) The number of tolerance phenotypes found per tag split into the ( c ) Bacteroidetes , ( d ) Proteobacteria and ( e ) Firmicutes phylums. The number of tags associated with each phylum is also reported ( n )=x. Full size image The distribution of the number of tolerance phenotypes linked to a specific tag varied widely. However, there were a large number of highly tolerant bacteria present. Indeed, 31% of the tags were linked to tolerance phenotypes towards all tested antibiotics ( Fig. 2b ). The recoveries of tags broadly resistant to antibiotics are most likely associated with highly abundant tags that could comprise several bacterial species. The taxonomic classification of the most tolerant tags highlighted that Porphyromonadaceae, Bacteroidaceae, Enterobacteriaceae and Enterococcaceae were the most tolerant taxa. Overall, the Lachnospiraceae and Ruminococcaceae carried the least tolerance along with a number of unclassified Firmicutes and unknown bacteria. This phylogenetic mapping of the antibiotic tolerance phenotypes allows a better understanding of the tolerance levels of specific taxonomic groups in the gut microbiota. For instance, many of our tolerant tags were classified as Bacteroides ( Bacteroidetes ; Fig. 2c ). Bacteria belonging to the phylum Bacteroidetes are among the most abundant in the human gut making up 20–30% of the total bacteria [9] . While there are some clinically relevant Bacteroides species (for example, Bacteroides fragilis ) they are generally considered as commensals or mutualists [37] . Interestingly, Bacteroides have previously been associated with antibiotic resistance transfer events [9] , [38] . In this study, we find that 39% of the tags belonging to Bacteroidetes are associated with pan-tolerance phenotypes, highlighting their potential as a reservoir of antibiotic resistance. Bacteria belonging to the phylum Proteobacteria , mostly Enterobacteriaceae , were also identified as highly tolerant in our sample. Enterobacteriaceae are of lower abundance in the gut, but the number of human pathogens and reports of resistance across classes of antibiotics associated with this group make it an important target of characterization [39] , [40] . Consistent with these reports [8] , we show that these tags are linked to tolerance towards most antibiotics tested ( Fig. 2d ). We also recovered many tags on the antibiotic selection plates that were not found on the control plates ( Supplementary Figs 7 and 8 ). These likely represent bacterial community members of lower abundance (representing minorities of the community) that may have been missed by insufficient sequencing depth or sampling. However, antibiotics capable of reducing or suppressing growth of abundant strains could select for these less abundant populations provided they could grow in the presence of the antibiotics. Among those drugs that recovered more rare tags were those that reduced the growth of highly abundant Bacteroidaceae ( Bacteroides ) and/or Enterobacteriaceae populations (erythromycin, sulfamethoxazole and ciprofloxacin; Supplementary Figs 7 and 9 ). These types of antibiotics could potentially be used to enrich cultivation for certain lower abundance populations of interest, as the medium itself was not the limiting factor in culturing these organisms. Indeed a previous study looking at the effect of ciprofloxacin treatment on human gut bacteria showed less perturbation in Lachnospiraceae and Clostridiales with treatment [41] , supporting our enrichment for these groups on ciprofloxacin plates. It should be noted that this technique is not able to distinguish between bacteria with intrinsic tolerance traits and transferable elements. Also, the association of a single tag with 15 tolerances does not mean that all bacteria with the same sequence carry all 15 tolerances. There are likely subpopulations of cells that only carry a fraction of the tolerance traits, but when looking at the total population of that particular tag, at least one cell has tolerance to each of the antibiotics where tolerance was observed. Population-based resistance mechanisms, as demonstrated in E. coli communities [42] , could also provide bacteria with protection from antibiotics without themselves carrying any tolerance traits. Recovery of uncultivated bacteria using phenotypic mapping To demonstrate the ability to enrich for subpopulations and recover specifically targeted taxa containing previously uncultured bacteria, a frozen sample of mixed bacteria preserved from antibiotic phenotyping plates (ciprofloxacin, sulfamethoxazole and erythromycin) and a fresh sample from the same human subject were anaerobically cultured on antibiotic selective media (Methods). Using the Human Microbiome Project’s Most Wanted List ( http://hmpdacc.org/most_wanted/ ) as a guide we tailored a combination of antibiotics based on the phenotyping data ( Supplementary Fig. 9 ) to select for those taxa listed, specifically targeting Odoribacter, Oscillibacter, Ruminococcus and Faecalibacterium ( Fig. 3a ). One hundred and ninety-two individual colonies were screened via 16S Sanger sequencing to determine their identity. A total of 106 sequences were retrieved with 26 unique isolates identified. Five of those isolates had 95% or less identity to previously cultured isolates ( Supplementary Data 5 ). 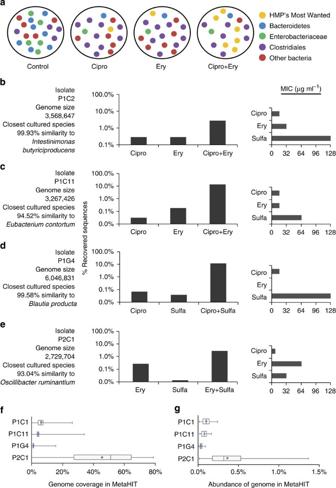Figure 3: Tailoring cultivation conditions allows recovery and characterization of specific bacteria. (a) The use of particular antibiotics (or combinations) helps select for the cultivation of bacteria of interest (previously uncultured and those on the Human Microbiome Project’s (HMP) Most Wanted List). Particular antibiotics (for example, Ciprofloxacin (Cip), Erythromycin (Ery), Sulfamethoxazole (Sulfa)) preferentially select for bacterial taxa that have few cultured isolates as compared with non-selection (Control). Combining antibiotics helps to further narrow the recoverable bacteria by exclusion of strains susceptible to both antibiotics. Therefore, particular combinations of drugs (for example, Cip and Ery) are able to increase the recovery of strains that belong to poorly cultured taxa (such as HMP’s Most Wanted List). (b–e) The four bacteria cultivated and genome sequenced based on multiplex phenotyping. The isolate name, genome size and closest similarity (16S) to a previously cultured bacterium are indicated. A graph of the percentage of bacteria from either a specific isolate (b,e) or the generaEubacterium(c) andBlautia(d) recovered on culture plates with a single antibiotic versus a combination of antibiotics demonstrates successful targeted recovery based on phenotyping data. The MIC data on ciprofloxacin, erythromycin and sulfamethoxazole tolerance for each of the four sequenced isolates is also reported. (f,g) The four genomes mapped to publically available MetaHIT metagenome data to determine their percentage genome coverage and abundance. For the box plots, the whisker bars span the minimum to maximum values, while the box defines the 1st quartile, the median and the 3rd quartile. The blue diamond denotes the mean. (f) The genome coverage represents the percentage of each of the four genomes that is covered by at least one read among MetaHIT metagenomes. (g) The abundance represents the total percentage of the metagenomes represented by each of the four sequenced genomes. Figure 3: Tailoring cultivation conditions allows recovery and characterization of specific bacteria. ( a ) The use of particular antibiotics (or combinations) helps select for the cultivation of bacteria of interest (previously uncultured and those on the Human Microbiome Project’s (HMP) Most Wanted List). Particular antibiotics (for example, Ciprofloxacin (Cip), Erythromycin (Ery), Sulfamethoxazole (Sulfa)) preferentially select for bacterial taxa that have few cultured isolates as compared with non-selection (Control). Combining antibiotics helps to further narrow the recoverable bacteria by exclusion of strains susceptible to both antibiotics. Therefore, particular combinations of drugs (for example, Cip and Ery) are able to increase the recovery of strains that belong to poorly cultured taxa (such as HMP’s Most Wanted List). ( b – e ) The four bacteria cultivated and genome sequenced based on multiplex phenotyping. The isolate name, genome size and closest similarity (16S) to a previously cultured bacterium are indicated. A graph of the percentage of bacteria from either a specific isolate ( b , e ) or the genera Eubacterium ( c ) and Blautia ( d ) recovered on culture plates with a single antibiotic versus a combination of antibiotics demonstrates successful targeted recovery based on phenotyping data. The MIC data on ciprofloxacin, erythromycin and sulfamethoxazole tolerance for each of the four sequenced isolates is also reported. ( f , g ) The four genomes mapped to publically available MetaHIT metagenome data to determine their percentage genome coverage and abundance. For the box plots, the whisker bars span the minimum to maximum values, while the box defines the 1st quartile, the median and the 3rd quartile. The blue diamond denotes the mean. ( f ) The genome coverage represents the percentage of each of the four genomes that is covered by at least one read among MetaHIT metagenomes. ( g ) The abundance represents the total percentage of the metagenomes represented by each of the four sequenced genomes. Full size image Genomic sequencing was performed on four of the 26 recovered isolates (two of those with identities of less than 95% to a cultured isolate) and MIC testing was done to confirm the previously collected phenotyping data ( Fig. 3b–e ). The effectiveness of combining antibiotics to selectively culture isolates of interest can be clearly demonstrated with the increased recovery of the targeted genera ( Eubacterium and Blautia ; Fig. 3c,d ) or strains (P1C2 and P2C1; Fig. 3b,e ) when antibiotic combinations are used versus single drugs. Genomic sequencing confirmed that two of these genomes had 16S rRNA identities of less than 95% to previously cultured bacteria suggesting they are likely to be new species. Isolates P1C2 and P1G4 had a high similarity (>99%) to previously cultured isolates Intestinimonas butyriciproducens and Blautia producta . Our novel isolates were most closely related to species Eubacterium contortum (94.8% similarity; P1C11) and Oscillibacter ruminantium (93% similarity; P2C1). The abundance of these isolates in the uncultivated library was very low or undetected ( Supplementary Table 2 ). RAST (ref. 43 ) annotations indicated that all bacteria carried multiple antibiotic resistance genes conferring resistance to aminoglycosides, streptothricin, vancomycin, tetracycline, beta-lactams, fluoroquinolones and multidrug efflux pumps. To assess the abundance of these new isolates in gut metagenomes, we mapped the reads from the publicly available MetaHIT [44] data to the sequenced genomes. We first determined what percentage of each of our genomes was covered in the MetaHIT samples and then quantified the overall abundance of the four genomes within the MetaHIT metagenomes ( Fig. 3f,g ). Isolates P1C2, P1C11 and P1G4 had low genome coverage and abundance among the MetaHIT data, which might suggest that they are of low abundance or these particular isolates are not ubiquitous to the human microbiome. However, our Oscillibacter -like isolate had a high percentage of coverage across the MetaHIT samples (43% average) and abundances of up to 1.36% in some metagenomes. Metagenomic data has suggested the existence of 19 species of Oscillibacter without a reference genome [45] . Genome comparisons in RAST of our Oscillibacter -like isolate (P2C1) with Oscillibacter ruminatium GH1, our Intestinimonas butyriciproducens isolate (P1C2), an unrelated gut microbe Bifidobacterium animalis subsp. lactis AD011 and a non-gut organism Geobacillus thermodenitrificans NG80-2 were undertaken to determine if there were any regions of high sequence homology between isolates ( Supplementary Fig. 10 ). Surprisingly, the I. butyriciproducens isolate had more regions of high homology than the O. ruminantium GH1 genome, but we are unable to speculate on the functional similarities as they were mainly hypothetical proteins. Uncultured Oscillibacter have been previously associated as responders to dietary change and as depleted in patients suffering from Crohn’s disease [46] , [47] . The ability to cultivate such organisms and study their physiology will contribute to our understanding of gastrointestinal disorders and devising treatment strategies. It is commonly believed that cultivation-based approaches are only able to capture a small part of organisms within the gut microbiota. Yet, our study has identified factors that can successfully help recover a representative fraction of the bacterial communities found in the human gut using techniques that can be readily implemented in most labs. Optimized cultivation procedures allow for multiplex mapping of phenotypes by directly coupling selective culture conditions with phylogenetic tag sequencing. In this way, we surveyed the prevalence of antibiotic phenotypes in the human gut microbiota. The tolerances can be directly linked to specific taxa and provide useful phenotypic information that cannot readily be derived from culture-independent studies. We sampled a substantial proportion of the cells (10 10 ) in the human gut microbiota and were able to identify both common and rare tolerances. In this way, we were able to detect a variety of taxonomic groups and assess the phylogenetic distribution of antibiotic tolerance phenotypes. Cultivation-based multiplex phenotyping is a quick and easy way to screen for antibiotic tolerance and look for tolerance patterns in human gut bacteria and should be a useful approach for studying the response to antibiotic treatment of the gut microbiome as well as illuminate possible risk factors predisposing individuals for antibiotic-associated diarrhoea and other diseases. Antibiotic tolerance phenotyping constitutes one useful application of cultivation-based multiplex phenotyping; however, this approach also has the potential to be used to identify substrate-specific utilization phenotypes as well as other tolerance phenotypes, including tolerance towards bile salts or high/low pH. This methodology could also be modified and applied to other environments such as soil or water to characterize phenotypic traits of interest. Notably, direct phenotyping can identify phenotypic characteristics, which cannot be as definitively characterized on a genetic basis and linked to specific bacteria using culture-independent methods. Finally, mapping the antibiotic tolerance profiles among bacteria in the gut allowed us to target the recovery of specific taxa with previously uncultured isolates. As a proof of concept, we identified four isolates, two of them novel species. One of these isolates appears to be a novel species of Oscillibacter ; uncultivated strains belonging to this genus are significantly reduced in patients suffering from Crohn’s disease. The ability to cultivate novel species with potential health benefits could be of interest to the probiotics industry and facilitate the development of novel probiotic supplements. Sample collection All faecal samples were collected from two healthy adult human donors that had not taken antibiotics in the past year. One donor (D1) supplied three samples (T1, T2, T3), while the other donor (D2) supplied four samples over time (T1, T2, T3, T4). Sample D1-T1 was utilized for the initial media culture comparison, samples D1-T2 and all D2 samples were used to confirm reproducibility of culturing results, sample D1-T2 was used for the antibiotic tolerance phenotyping, and samples D1-T2 (frozen cultivated sample) and D1-T3 for directed recovery of bacteria. Consent was gained from all participants and proper ethical guidelines (Hvidovre Hospital) were followed throughout the study. Samples were transported to an anaerobic chamber within 5 min of collection. Five grams was separated out for culturing and 2.5 g was collected for total DNA extractions. The remaining sample was stored at −80 °C. Media The complete compositions of all media are listed in the Supplementary Methods . Cultivation, viable cell counts and DNA extraction All manipulations were performed in a Type B Vinyl Anaerobic Chamber (Coy Lab Products) filled with an atmosphere of 95% nitrogen and 5% hydrogen. Five grams of faecal sample was homogenously resuspended in 50 ml of 1 × PBS that had been pre-reduced with resazurin (0.1 mg ml −1 ). Ten-fold serial dilutions were performed to 10 −9 . Fifty microlitres of the 10 −3 , 10 −4 and 10 −5 dilutions were combined in equal proportion with 0.4% trypan blue. The countable dilution was identified and a hemocytometer and light microscope were used to perform a viable cell count in the anaerobic chamber. Viable cells counts were done in triplicate for each sample (per time point), and viable counts were performed three separate times for the same individual to make sure that recovery counts were consistent over time. The samples utilized for the viable cell counts included D1-T1, D1-T2, D1-T3, D2-T1, D2-T2 and D2-T3. Total cell counts were also performed on two samples from D1 to determine the fraction of cells that were not viable and/or culturable. We never observed the culturable cells as a higher number than the viable or total cells. One hundred microliters of the serial dilutions were plated in five replicates on each of the 10 media ( Supplementary Methods ) to be tested. Seven to 12 sterile glass beads were used to spread the liquid on the plates through even shaking. Plates were anaerobically incubated at 37 °C for 7 days. Plate counts were conducted each day to track the growth over time. On day 7, three dilutions, consisting of the countable dilution (between 25 and 250 colonies) and the dilutions above and below it, were chosen to select for a variety of plate crowding conditions (exceptions occurred for the Minimal and GMM media, where four dilutions were collected to accommodate lower overall plate counts). None of the plate dilutions utilized represented a situation where a lawn was formed or the plate would not be able to be counted. While it is not possible to confirm that all colonies scraped off the plates grew as individual colonies rather than co-cultures, the visual observations of the plates indicated that most colonies did not appear to touch. Further evidence to support this observation is that 95% of the individual colonies picked into 96-well plates (see below) from dilution plates resulted in the identification of a single species. These dilutions were manually scraped off the media surface following a rinse with 5 ml 1 × PBS and collected into 10 ml tubes. The collected tubes were centrifuged at 5,000 g for 30 min and remnants of solid media were carefully removed from the pelleted samples. The pelleted samples were then extracted as individual dilutions (except Minimal and some GMM dilutions) using the MoBio UltraClean Microbial DNA Isolation kit. The uncultivated total faecal sample was extracted using 2.5 g of sample and the MoBio PowerMax Mega Soil DNA Isolation kit. PCR and sequencing Extracted DNA was diluted to 5 ng μl −1 for all samples in order to keep quantities constant for the amplification step. PCR was performed using 1 × Phusion High-Fidelity PCR Master Mix and tagged Illumina primers (10 μM concentration) in 30 μl reactions targeting the hypervariable V6 region (positions 969–1,046; primer and barcode sequences listed in Supplementary Data 6 ). Illumina overhangs (100 μM concentration) were attached in a second PCR reaction by combining barcoded samples in equal amounts as template for amplifying multiple 30 μl reactions. Thermocycling conditions for both PCR steps were as follows: initial denaturation 98 °C for 1 min, followed by 30 cycles of 98 °C for 10 s, 65 °C for 30 s and 72 °C for 30 s, and a final elongation at 72 °C for 5 min. PCR product sizes were confirmed at each step and the final PCR product was gel purified using the Qiaex II Gel Extraction Kit (Qiagen). The samples were sequenced on an Illumina MiSeq. Sequence quality control and processing Sequence quality control, processing and analysis was performed using a modified version of the sequence quality control and analysis protocol [48] recommended for mothur (version 1.30.2) (ref. 49 ). To pass the initial quality control, the sequence needed to (i) perfectly match the barcode, forward primer and last 15 bases of the reverse primer, (ii) have a rolling window quality of 30 (rolling window size of 25); the sequences were truncated where they fell below quality window (iii) contain no ambiguous bases, (iv) have homopolymers of no more than eight bases and (v) have a minimal length of 60 bp (refs 28 , 48 , 50 ). Sequences that did not align along the same region (full V6) based on the Silva alignment were removed from the analysis. Sequences only occurring a single time (more than 50% of the unique sequences) were removed following the alignment step to denoise and reduce the dataset for further processing. The reverse primer and all but four bases of the forward primer were removed from the sequences. The four bases of the forward primer were kept as a reference to confirm correct alignment throughout the analysis. A pre-clustering step in mothur (1 bp difference) was performed as recommended to reduce tag number inflation due to sequence errors [51] . Samples were checked for chimeras using Uchime [52] and sequences identified as non-bacterial or unknown (80% cutoff) were removed from further analysis. Sequences were then compared at a 0% difference (unique) cutoff, giving each unique sequence its own taxonomic signature, which we refer to as a ‘tag’. Sequences from multiple dilutions recovered from each media type were combined in equal proportions to better represent recovery from each media; for example, the sequences from the 3 GM5 dilutions (D5, D6, D7) were combined in equal proportion to represent the GM5 media. For each group of samples analysed together, the sequences were sub-sampled (36,040 for media comparison and 15,450 for antibiotic phenotyping) to equalize the number of sequences per sample and rare sequence removal cutoff was established at 0.0166% abundance (abundance of five or less for 30,000 sequences). Total tags and Morisita–Horn indices were calculated in mothur. BIOM files created in mothur were exported to MEGAN [53] to visualize taxonomic classifications on a family level and taxonomic classification and abundances as defined in mothur were used to construct further taxonomic graphs. Sequence abundance data and taxonomic classifications were used to create heat maps in R. Culturing of antibiotic tolerant bacterial community One hundred microliters of the serial dilutions were plated in two replicates on GM7 agar containing one of the 16 antibiotics. The GM7 medium was chosen for the antibiotic tolerance testing because samples cultivated on this medium showed good similarity to the uncultivated sample and because gellan-containing media has not yet been shown effective for antibiotic susceptibility testing. The selected antibiotic concentrations were based on Eucast data ( http://mic.eucast.org/Eucast2/ ) of commensal gut bacteria, (mostly Bacteroidetes, Enterococcaceae, Enterobacteriaceae and Lactobacillus ), and were aimed for 2 × higher than MICs ( Supplementary Fig. 5 ). Seven to 12 glass beads were used to spread the liquid on the plates through even shaking. Plates were anaerobically incubated at 37 °C for 5 days. These dilutions were manually scraped off the media surface following a rinse with 5 ml 1 × PBS and collected into 10 ml tubes. One ml of the collected sample was centrifuged at 5,000 g for 30 min and remnants of the solid media were carefully removed from the pelleted samples. DNA was then extracted from pelleted samples using the MoBio UltraClean Microbial DNA Isolation kit. The remaining 9 ml of the collected colonies was preserved at −80 °C in 10% glycerol stocks. Anaerobic cultivation of new bacterial isolates Frozen stocks of bacterial colonies (100 μl) previously scraped off ciprofloxacin, sulfamethoxazole and erythromycin plates were plated in duplicate serial dilutions on GM7 media containing either erythromycin or sulfamethoxazole (concentrations as above). A fresh faecal sample from the same subject was used to make serial dilutions in duplicate on erythromycin and control (no antibiotics) plates. Plates were incubated anaerobically at 37 °C for 5 days. Ninety-six colonies from the frozen samples and 96 colonies from the fresh sample were freshly isolated on new media. Colony PCR was performed on the 16S rRNA region for the two 96-well plates using primers 8F (5′-AGAGTTTGATCCTGGCTCAG-3′) and 1391R (5′-GACGGGCGGTGTGTRCA-3′) and Sanger sequenced using the forward primer. The sequences were quality control processed in CLC Main Workbench, and BLAST [54] and EzBioCloud [55] were used to identify the sequences. A total of 26 unique sequences were identified and the closest match to a cultured reference sequence was determined ( Supplementary Data 5 ). Genome sequencing, processing and analysis Bacteria to be genome sequenced were anaerobically grown up in GAM broth for 1–3 days at 37 °C. DNA from these bacteria was isolated using the MoBio UltraClean Microbial DNA Isolation Kit, genome sequence libraries were constructed using the Nextera DNA Sample Preparation Kit and sequencing was performed on an Illumina MiSeq (150 bp paired-end reads). Genome assembly was done using Velvet (v1.09) (ref. 56 ), and contigs that were less than 500 bp or with less than 3X coverage were filtered. The range of kmer values used were 93–125, and the assembly providing the best N50 score was used. Annotation of the assembled genomes was done using RAST (ref. 43 ). RAST was also used to generate genome sequence comparisons between several isolates and publically available genomes. In addition, the high-quality reads from the MetaHIT project [44] were aligned to each of the assembled genomes. Read alignment was done using Bowtie2 (v2.1.0) (ref. 57 ), with processing of the alignment files was done using SAMTools (v0.1.19) (ref. 58 ). Coverage and sequencing depth of the aligned reads was assessed using BEDTools (v2.17.0) (ref. 59 ). The abundance of each assembled genome in the MetaHIT samples was calculated as the number of reads that aligned to the genome divided by the total number of reads. Accession codes : Sequence reads for the 16S rRNA amplicon sequences have been deposited in the NCBI Sequence Read Archive under the BioSample code SAMN02869573, within BioProject PRJNA253252. The full 16S nucleotide sequences from the cultured isolates have been deposited in the GenBank NCBI nucleotide database with accession codes KM043745 to KM043770. The genome sequences were deposited in the NCBI Whole Genome Shotgun database under accession codes JPJD00000000, JPJE00000000, JPJF00000000 and JPJG00000000, within BioProject PRJNA253252. How to cite this article: Rettedal, E. A. et al. Cultivation-based multiplex phenotyping of human gut microbiota allows targeted recovery of previously uncultured bacteria. Nat. Commun. 5:4714 doi: 10.1038/ncomms5714 (2014).